Amerindian-specific regions under positive selection harbour new lipid variants in Latinos Dyslipidemia and obesity are especially prevalent in populations with Amerindian backgrounds, such as Mexican–Americans, which predispose these populations to cardiovascular disease. Here we design an approach, known as the cross-population allele screen (CPAS), which we conduct prior to a genome-wide association study (GWAS) in 19,273 Europeans and Mexicans, in order to identify Amerindian risk genes in Mexicans. Utilizing CPAS to restrict the GWAS input variants to only those differing in frequency between the two populations, we identify novel Amerindian lipid genes, receptor-related orphan receptor alpha (RORA) and salt-inducible kinase 3 ( SIK3 ), and three loci previously unassociated with dyslipidemia or obesity. We also detect lipoprotein lipase (LPL) and apolipoprotein A5 ( APOA5 ) harbouring specific Amerindian signatures of risk variants and haplotypes. Notably, we observe that SIK3 and one novel lipid locus underwent positive selection in Mexicans. Furthermore, after a high-fat meal, the SIK3 risk variant carriers display high triglyceride levels. These findings suggest that Amerindian-specific genetic architecture leads to a higher incidence of dyslipidemia and obesity in modern Mexicans. Dyslipidemia is a highly prevalent (53%) [1] cardiovascular risk factor in the United States that will drastically increase medical and economic burdens in the subsequent decades if prevention and treatment cannot be better tailored for those most susceptible. In addition to socioeconomic status, the prevalence of lipid disorders also varies among ethnic groups, with Hispanics being more prone to dyslipidemia than any of the other US groups [2] . With 40% of Mexican–American men and 35% of women exhibiting high triglycerides (TGs) (>1.69 mmol l −1 ) [2] , a large portion of the population has a high risk of cardiovascular disease (CVD), especially as a direct causal relationship between hypertriglyceridemia and CVD was recently demonstrated [3] . Strikingly, the decreasing rate of CVD currently observed in Europeans [4] does not extend to Hispanic-origin populations, as exemplified by the four times higher incidence of CVD among the Amerindians when compared with Europeans [2] . Thus, identifying Hispanic-specific lipid variants is critical to deciphering the genetic pathogenesis of dyslipidemia and CVD in this rapidly growing US minority, and ultimately personalizing prevention and treatment of this major risk factor. Despite their increased predisposition [5] , Mexicans and other groups with Amerindian heritage have been substantially underrepresented in genomic studies [6] , [7] . Most lipid studies focus on recapturing European-origin signals in the Latino populations [8] , [9] , [10] , [11] , [12] , [13] , with only a single Mexican lipid genome-wide association study (GWAS) reported [14] . GWAS in admixed populations are hindered by a complex population substructure that can reduce power [15] . Statistical methods, such as local ancestry inference or admixture mapping, have been employed to overcome or even utilize such ancestral variations to identify disease-associating loci in diverse populations; however, they often rely on ancestry-informative markers or parental population haplotype panels that are not readily available in all populations, as is the case with Latinos [16] , [17] , [18] . Fitting a mixed model or adjusting for ancestry in GWAS can circumvent the confounding effect of ancestry, but may lead to a higher false-negative rate and losing ancestry-specific variants [14] , [15] . To this end, we design an approach utilizing cross-population allele screen prior to GWAS (CPAS-GWAS) to identify Amerindian-origin lipid variants in Mexicans. Utilizing the CPAS-GWAS approach, we identify 18 Amerindian risk variants for lipids and obesity and one risk haplotype for TGs in Mexicans. Interestingly, the Amerindian-specific TG risk haplotype and 10 of the Amerindian lipid and obesity variants have not been implicated in lipid traits or obesity in other populations. Two of the new TG loci also show signs of potential positive selection, reflecting the possibility that maintaining high serum lipid levels was favourable during the Amerindian population history. Accession codes : The Mexican hyperTG case-control GWAS data have been deposited in NIH dbGAP database under the accession code phs000618.v1.p1. A novel cross-population allele screen approach To search for Amerindian-specific genetic variants that contribute to the high risk of dyslipidemia and obesity in Mexicans, we developed a CPAS-GWAS approach that first screens across the genome for variants that differ in frequency between the two ancestry populations, Europeans and Amerindians, and subsequently includes only these variants (CPAS variants) in the actual Mexican GWAS. Thus, we restricted the Mexican GWAS to variants only present in Mexicans and not in Europeans, and variants that show statistically significant differences in allele frequency between Mexicans and Europeans, as explained in detail below (see Supplementary Fig. 1 for CPAS design). CPAS enriches for Amerindian TG variants We first screened for population-specific variants between the admixed Mexican population and its European ancestry population represented by Finns, using Finnish and Mexican controls matched on the tested phenotype (that is, Finns and Mexicans with normal levels of TGs, total cholesterol (TC), high density lipoprotein cholesterol (HDLC) or body mass index (BMI), respectively). The purpose of the phenotypic matching is to ensure that the differences in allele frequencies are strictly due to population structure in order to focus on the variants that are population-stratified instead of confounded by other phenotypes. Based on our local ancestry estimates, African ancestry is low (2.3%) in the Mexican cohort, and accordingly, no screening between Mexican and African controls was performed. For screening across the genome, we first imputed the GWAS data in the Finnish and Mexican cohorts to increase both the number of overlapping common variants between the cohorts and the number of low-frequency single-nucleotide polymorphisms (SNPs) (minor allele frequency (MAF) 1-5%), known to differ most between populations [19] . Overlapping SNPs with MAF>5% in Mexicans were pruned using an R 2 cutoff of 0.5 in the Mexican controls to reduce redundancy and multiple testing. To avoid overestimation of linkage disequilibrium (LD) among the low-frequency variants, all overlapping SNPs with MAF 1–5% in Mexicans were retained. In the actual TG CPAS screen, 967,056 SNPs (61%) exhibited a difference in allele frequencies between Mexican and Finnish TG controls that passed the Bonferroni correction ( P <3.16 × 10 −16 ) for 1,584,455 SNPs tested. A Mantel–Haenszel test showed that the MAF distribution difference is significantly greater between populations after CPAS ( P <2.20 × 10 −16 ), indicating that population-stratified variants were indeed detected ( Fig. 1a,b ). In addition, we compared these variants between Europeans and admixed Native Americans from the 1000 Genomes Project, and 74% of them displayed >10% difference in MAF, demonstrating that our screening does filter for variants that differ between the populations. We also included in the GWAS the 694,185 Mexican-specific SNPs that after imputations were only present in Mexicans but not in Finns to further enrich the GWAS for Amerindian-specific variants. Taken together, 1,661,241 CPAS SNPs filtered by CPAS to significantly differ between Finns and Mexicans or not present in Finns were carried forward for association testing between Mexican TG cases and controls. CPAS was also carried out for three additional traits, HDLC, TC and BMI in a similar way. 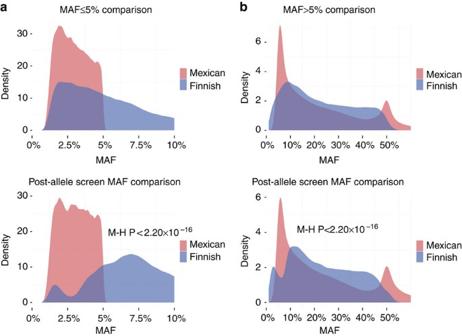Figure 1: Minor allele frequency distributions in the Finnish and Mexican low TG controls before and after the cross-population allele screen. (a) Displays the SNPs with a MAF≤5% in the Mexicans. These SNPs with a MAF≤5% were not pruned based on LD. (b) shows the SNPs with a MAF>5% in the Mexicans. These SNPs with a MAF>5% were pruned based on LD in the Mexican controls using anR2cutoff of 0.5. Mantel–Haenszel (M–H)P-value is displayed, indicating that the difference between the Mexican and Finnish frequencies was significantly different after the screen, and therefore, population-stratified variants are enriched due to the CPAS. Figure 1: Minor allele frequency distributions in the Finnish and Mexican low TG controls before and after the cross-population allele screen. ( a ) Displays the SNPs with a MAF≤5% in the Mexicans. These SNPs with a MAF≤5% were not pruned based on LD. ( b ) shows the SNPs with a MAF>5% in the Mexicans. These SNPs with a MAF>5% were pruned based on LD in the Mexican controls using an R 2 cutoff of 0.5. Mantel–Haenszel (M–H) P -value is displayed, indicating that the difference between the Mexican and Finnish frequencies was significantly different after the screen, and therefore, population-stratified variants are enriched due to the CPAS. Full size image GWAS results and independent replication We performed GWAS for high TGs in Mexicans using only the CPAS SNPs as the input. HDLC, TC and BMI were analysed as continuous traits instead to demonstrate that CPAS-GWAS is effective for quantitative traits as well. As the four phenotypes are highly correlated, we only corrected for the number of SNPs using Bonferroni in the GWAS step, followed by the replication step in which we also corrected for multiple testing using Bonferroni. The top 1% of the TG GWAS results are shown in Supplementary Data 1 . We selected 15 non-redundant TG SNPs with P -values 1.07 × 10 −5 −6.08 × 10 −33 for replication in 6,159 additional Mexican individuals based on P -value, functional annotation and MAF difference between Mexicans and Finns ( Table 1 and Supplementary Table 1 ). Three of the 15 SNPs were Mexican-specific as their frequencies were less than 1% in the Finnish cohort or Europeans (the 1000 Genomes database). 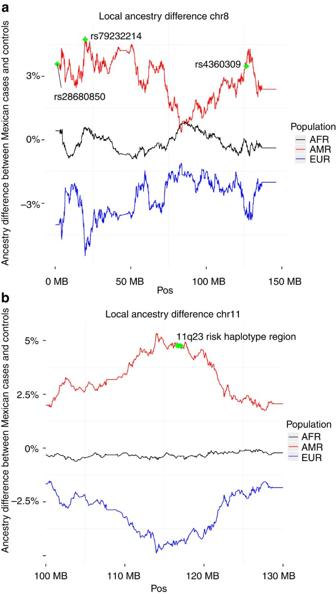Figure 2: Local ancestry difference between Mexican low TG controls and high TG cases in the genomic regions implicated by the CPAS-GWAS. (a) Local ancestry results are shown for chromosome 8. Rs28680850 and rs79236614 were both significant after Bonferroni correction and rs4360309 displayed a suggestive signal in the GWAS. All three variants reside in regions that show Amerindian enrichment in Mexican high TG cases (>3% Amerindian ancestry difference). (b) Local ancestry difference between Mexican low TG controls and high TG cases on chromosome 11q23 where the TG risk haplotype region resides. The seven haplotype-tagging SNPs are shown as green diamonds that are clustered together in the plot. These LAMP-LD17results indicate that the 11q23 region is highly enriched for Amerindian ancestry in the Mexican high TG cases. The Mexican replication sample ( n =6,159) consisted of an unrelated cohort and a family-based cohort (see Supplementary Table 2 for clinical characteristics). We combined the results from the two replication cohorts by performing a meta-analysis using METAL [20] . Table 1 CPAS-GWAS and replication results for case-control comparison of TGs. Full size table Four variants (rs28680850, rs79236614, rs964184 and rs139961185) on chromosomes 8 and 11 resulted in P -values less than the Bonferroni correction significance level ( P <0.0033) in the replication stage ( Table 1 ). Furthermore, their overall meta-analysis in all Mexican cohorts (GWAS combined with the replication cohorts, total n =9,482) resulted in P -values between 7.1 × 10 −9 −1.8 × 10 −67 . Interestingly, the intergenic variant rs79236614 that resides ~100 kb downstream of the lipoprotein lipase ( LPL ) gene is in high LD ( R 2 =0.91) in Mexicans with an early stop variant in LPL , rs328 (S474X), that cuts off the last exon ( Table 1 ). The novel TG variant rs28680850 on chr8p21 resides in a predicted CpG site. We verified its allele-specific effect on methylation by pyrosequencing bisulphite-treated whole blood-derived DNA samples from Mexicans. The homozygous individuals with the rs28680850 A risk allele ( n =11) all had a 0% methylation status, whereas individuals with AG and GG genotypes ( n =48) had a methylated CpG site with an average methylation of 57% (range 36–100%), implicating potential epigenetic regulation of TG levels. The new TG-associated variant on chr11, rs139961185 that resides in an intron of salt-inducible kinase 3 ( SIK3 ), is common in Mexicans but not observed in Finns ( Table 1 ). To eliminate the possibility that the association signal came from a correlation with the nearby, known TG-associated gene, apolipoprotein A5 ( APOA5 ), we carried out a regional LD analysis ( Supplementary Fig. 2 ). We did not observe any pair-wise R 2 >0.2 between rs139961185 and any of the APOA5 or APOC3 variants, indicating that this novel Mexican-specific TG variant in SIK3 is independent from APOA5 and APOC3 . In addition, four other SNPs (rs62436827, rs4360309, rs72925845 and rs78536982) showed suggestive TG signals ( P <0.05) in replication for the same allele and direction as in the GWAS ( Table 1 ). Six HDLC variants and three TC SNPs passed the genome-wide significance threshold ( P <5 × 10 −8 ) in the Mexican CPAS-GWAS ( Table 2 ). Two HDLC hits (rs78557978 and rs148533712) and the top BMI signal (rs6027281) that reside near novel genes that have never been implicated for these traits were selected for replication. HDLC and TC variants near or in known lipid genes such as CETP and CELSR2 were not selected for replication. Two novel HDLC loci, an intronic variant in receptor-related orphan receptor alpha ( RORA ) (rs148533712) and an intergenic variant near UDP glycosyltransferase 8 (rs78557978) were replicated ( Table 2 ). Since a known HDLC-associated gene, hepatic lipase ( LIPC ), is 2.3 Mb away from rs148533712, we performed a regional LD analysis ( Supplementary Fig. 3 ) to investigate whether this Mexican HDLC signal is independent from LIPC . The regional LD analysis demonstrated that the LD (in R 2 ) decays drastically before reaching LIPC , and there was no strong LD between rs148533712 and any variant within LIPC ( R 2 <0.2), indicating that the Mexican HDLC signal in RORA is independent from the previously known European LIPC lipid signal, as is also suggested by the relative long distance of 2.3 Mb. Interestingly, the associated interval around the latter SNP rs78557978 ( R 2 >0.5) includes only one gene, UDP glycosyltransferase 8. The replicated BMI hit, rs6027281 ( Table 2 ) resides between C20orf197 and LOC284757 . However, the associated interval ( R 2 >0.5) does not extend to these adjacent predicted genes, suggesting an intergenic regulatory effect for this BMI hit or its proxy. Table 2 CPAS-GWAS and replication results for quantitative lipid traits and BMI. Full size table TG CPAS-GWAS loci are enriched for Amerindian ancestry To provide additional support for our CPAS approach, we compared the four replicated TG signals with regions displaying enriched Amerindian ancestry in Mexican TG cases versus controls identified by using LAMP-LD [17] . Figure 2a,b shows that the four replicated TG variants reside in regions with the highest Amerindian ancestry difference across the whole genome (a percent difference>3% and a z -score>3 for an ancestry enrichment between the Mexican TG cases and controls). Supplementary Figs 4–6 show the close-up views of these loci with regional genes. Furthermore, three (rs78536982, rs72925845, and rs4360309) of the four suggestive loci also reside in regions with Amerindian enrichment (a percent difference >2%) in Mexican high TG subjects ( Supplementary Figs 7 and 8 ). Genome-wide ancestry difference is shown in Supplementary Fig. 9 . Figure 2: Local ancestry difference between Mexican low TG controls and high TG cases in the genomic regions implicated by the CPAS-GWAS. ( a ) Local ancestry results are shown for chromosome 8. Rs28680850 and rs79236614 were both significant after Bonferroni correction and rs4360309 displayed a suggestive signal in the GWAS. All three variants reside in regions that show Amerindian enrichment in Mexican high TG cases (>3% Amerindian ancestry difference). ( b ) Local ancestry difference between Mexican low TG controls and high TG cases on chromosome 11q23 where the TG risk haplotype region resides. The seven haplotype-tagging SNPs are shown as green diamonds that are clustered together in the plot. These LAMP-LD [17] results indicate that the 11q23 region is highly enriched for Amerindian ancestry in the Mexican high TG cases. Full size image Genome-wide SKAT analysis supports replicated TG loci To utilize the imputed low-frequency variants that are more likely to be population-specific [19] , we examined the combined effect of common and rare variants using combined sum test with sequence kernel association test (SKAT-C) analysis [21] . Only the CPAS SNPs were included as input variants in the SKAT-C. Both 11q23 and 8p21 loci where three (rs964184, rs139961185 and rs79236614) of the replicated SNPs from the single-marker analysis reside were significant in SKAT-C ( P <7.64 × 10 −7 ) after correcting for 65,428 regions tested ( Supplementary Fig. 10a–c ). An additional peak near LPL with no GWAS hits is likely due to a cluster of regional rare variants driving the signal ( Supplementary Fig. 10a ). The 8p23.3 region where the fourth replicated GWAS SNP rs28680850 resides resulted in a suggestive SKAT-C P -value of P =2.70 × 10 −5 ( Supplementary Fig. 10b ). These results indicate that the use of CPAS variants in SKAT helps identify regions with population-based combined effects of common and rare variants. A mexican-specific TG risk haplotype We observed a well-known TG- and coronary heart disease (CHD)- associated locus on chromosome 11q23 [8] , [9] , [10] , [11] , [12] , [13] , [14] , [22] in three separate analyses, CPAS-GWAS, LAMP-LD ( Fig. 2b ), and CPAS-SKAT ( Supplementary Fig. 10c ), with rs964184 showing the strongest genome-wide signal for TGs ( P =6.08 × 10 −33 ) ( Table 1 ). Interestingly, 15 additional non-redundant CPAS variants ( R 2 <0.5), all within 500 kb of the lead SNP rs964184, produced P -values of 5.77 × 10 −7 −1.58 × 10 −16 in the GWAS, four of these were Mexican specific (European MAF<1%). When conditioned on rs964184, the 15 SNPs were no longer associated ( P >0.05) (see Supplementary Data 2 for a detailed LD structure among these SNPs). This raised the possibility of a TG-associated, Mexican-specific haplotype on chr11. To investigate this issue, we performed the LD analysis using D′. All 15 SNPs showed high D′ (>0.5) with rs964184, and a haplotype association analysis of these 16 SNPs resulted in an overall P -value of 1.04 × 10 −16 between the Mexican TG cases and controls. Consequently, we identified a 460-kb TG-associated risk haplotype (HT1) formed by seven SNPs ( Fig. 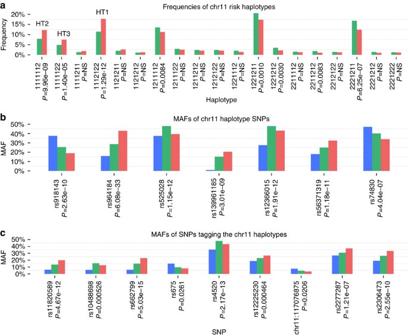Figure 3: Frequencies of the chr11 haplotypes and variants in the TG risk region. (a) Frequencies of chr11 risk haplotypes between the Mexican TG cases and controls. TheP-value of the omnibus haplotype was 1.93 × 10−24using the haplotype case/control test in PLINK. Red bars represent the haplotype frequencies in the Mexican cases and green bars the frequencies in the Mexican controls. NS indicates nonsignificant (P>0.05). The order of the SNPs on the haplotype is rs918143 (1/C), rs964184 (1/G), rs525028 (1/G), rs139961185 (2/A), rs12366015 (1/A), rs56371319 (2/A) and rs74830 (2/T) with the TG-increasing allele given in parenthesis. (b) The minor allele frequencies of the seven haplotype SNPs in the order of Finnish TG controls, Mexican TG controls and Mexican TG cases. (c) The minor allele frequencies of the nine SNPs travelling with the two chr11 risk haplotypes in the same order of groups as inFig. 3babove. 3a , Supplementary Table 3 ) with a haplotype frequency of 18% in Mexican TG cases (overall haplotype P =1.93 × 10 −24 and the risk haplotype P =1.29 × 10 −12 ) ( Supplementary Table 3 ). The two other TG-increasing haplotypes (HT2 and HT3) resulted in P -values of 9.96 × 10 −9 and 1.40 × 10 −5 ( Supplementary Table 3 ). Figure 3b shows the MAFs of the seven haplotype SNPs in the Finns and Mexicans. Figure 3: Frequencies of the chr11 haplotypes and variants in the TG risk region. ( a ) Frequencies of chr11 risk haplotypes between the Mexican TG cases and controls. The P -value of the omnibus haplotype was 1.93 × 10 −24 using the haplotype case/control test in PLINK. Red bars represent the haplotype frequencies in the Mexican cases and green bars the frequencies in the Mexican controls. NS indicates nonsignificant ( P >0.05). The order of the SNPs on the haplotype is rs918143 (1/C), rs964184 (1/G), rs525028 (1/G), rs139961185 (2/A), rs12366015 (1/A), rs56371319 (2/A) and rs74830 (2/T) with the TG-increasing allele given in parenthesis. ( b ) The minor allele frequencies of the seven haplotype SNPs in the order of Finnish TG controls, Mexican TG controls and Mexican TG cases. ( c ) The minor allele frequencies of the nine SNPs travelling with the two chr11 risk haplotypes in the same order of groups as in Fig. 3b above. Full size image Logistic regression of the TG case/control status on the HT1 haplotype carrier status resulted in OR=1.65 ( P =7.79 × 10 −14 ), suggesting that HT1 is a significant risk factor for high TGs in Mexicans. Interestingly, HT1 is Mexican-specific and not observed in Finns, because it is tagged by rs964184 and rs139961185 ( Supplementary Table 3 ) of which rs139961185 is Mexican-specific (not observed in Finns and MAF=0.5% in the 1000 Genomes Europeans). This Mexican-specific risk HT1 also showed strong association with high TGs in the replication cohorts ( P =7.09 × 10 −12 , OR=1.46) with a frequency of 20% in the Mexican TG cases (overall haplotype P =2.83 × 10 −41 and the risk haplotype P =2.51 × 10 −13 ). Two causative TG variants on the haplotype background To identify causative variants travelling on the haplotype background, we examined all SNPs in the haplotype region, focusing on the Mexican-specific HT1. Eight exonic SNPs on the HT1 background, as well as one known hypertriglyceridemia promoter SNP [14] , [23] on the HT2 background, were further investigated based on differences in allele frequencies and potential deleterious effect ( Fig. 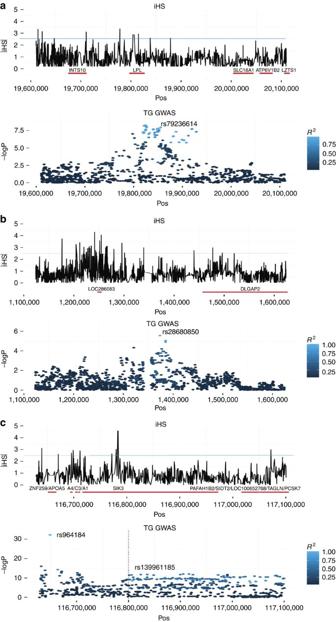Figure 4: Analysis of natural selection in the three Mexican TG risk regions. The absolute |iHS| were plotted across the three TG risk loci in the upper panel. A blue line indicates the top 1% chromosome-wide |iHS| threshold (>2.56). For comparison, the lower panel shows the logistic regression results of the Mexican TG case/control sample for the same SNPs (MAF>5%) in each region. LD (inR2) is plotted against the regional lead SNP. All 3,701 Mexican individuals were included in the iHS analysis. (a) The |iHS| results on chr8p21. The highest peak was observed in theLPLpromoter region although no extreme |iHS| scores (>4) were observed. (b) The |iHS| results on chr8p23.3. A region harbouring a lincRNA,LOC286083shows signs of positive selection with peaks of extreme |iHS| values. (c) The |iHS| results of chr11q23. Clusters of extreme |iHS| scores in theSIK3region suggests that it underwent positive selection pressure in Mexicans. In the lower panel, LD is measured against rs964184 or rs139961185, respectively, before or after the 168 MB bp position, indicated by the vertical line. 3c ; Supplementary Table 4 ). To identify variants that best explain the Mexican TG case/control status, we carried out a step-wise logistic regression including all nine SNPs. Rs11820589 and rs662799 were retained in the model ( P <0.00001; Fig. 3c ) with a pseudo- R 2 value of 0.057, indicating that these SNPs tagged by the risk haplotypes explain ~6% of high TG levels in the Mexican cohort. Interestingly, rs11820589 is in LD ( R 2 =0.82) with a known non-synonymous variant, rs3135506 in APOA5 (ref. 24 ). A PolyPhen 2 score of 0.993 and a SIFT score of 0 for rs3135506 indicate a possible damaging effect on the protein. Thus, a change in TGs attributed to rs11820589 is likely due to the effect of rs3135506 on APOA5 . Based on ENCODE data, rs662799 (2 kb upstream of APOA5 ) is a strong enhancer in a HepG2 liver cell line, probably regulating APOA5 in cis , as APOA5 is highly expressed in liver. In summary, these two variants explain ~6% of TG levels in Mexicans likely due to a change of function of APOA5 . Positive selection on Amerindian TG loci To examine if the top TG GWAS loci were favourably retained in the Mexican population due to recent positive natural selection, we examined the integrated haplotype score (iHS) statistics of neutrality (see Methods) for all genotyped and imputed SNPs with MAF>5% across the chr8 and chr11 regions ( Fig. 4 ) instead of just the CPAS variants, because focusing only on the CPAS variants that differ in allele frequency between the two populations would have introduced a bias into our selection analysis [25] . In our selection analysis, we found multiple peaks of extreme |iHS| values (>4.0) in the chr11 risk haplotype region within the SIK3 gene ( Fig.4c ). It is worth noting that both the Mexican-specific, TG-associated haplotype-tagging SNP, rs139961185 and the novel Mexican-specific HDLC-associated variant rs11216230 also reside in SIK3 ( Tables 1 and 2 ). We estimated that these extreme |iHS| scores in SIK3 rank among the top 0.1% chromosome-wide scores based on our iHS analysis on all genotyped SNPs on the entire chr11, suggesting that SIK3 has been under recent positive selection and thus retained unusually high homozygosity. We also identified peaks with |iHS| >4.0 near the novel TG variant on chr8, residing inside a lincRNA gene, LOC286083 , expressed in most human tissues ( Fig. 4b ). The LPL region resulted in several |iHS| values >3.0, although no extreme |iHS| scores (>4.0) were seen in this TG region ( Fig. 4a ). Interestingly, the extreme iHS scores were observed with imputed SNPs, suggesting that the genotype panel does not represent well Mexican-specific variants and Latino populations in general. Figure 4: Analysis of natural selection in the three Mexican TG risk regions. The absolute |iHS| were plotted across the three TG risk loci in the upper panel. A blue line indicates the top 1% chromosome-wide |iHS| threshold (>2.56). For comparison, the lower panel shows the logistic regression results of the Mexican TG case/control sample for the same SNPs (MAF>5%) in each region. LD (in R 2 ) is plotted against the regional lead SNP. All 3,701 Mexican individuals were included in the iHS analysis. ( a ) The |iHS| results on chr8p21. The highest peak was observed in the LPL promoter region although no extreme |iHS| scores (>4) were observed. ( b ) The |iHS| results on chr8p23.3. A region harbouring a lincRNA, LOC286083 shows signs of positive selection with peaks of extreme |iHS| values. ( c ) The |iHS| results of chr11q23. Clusters of extreme |iHS| scores in the SIK3 region suggests that it underwent positive selection pressure in Mexicans. In the lower panel, LD is measured against rs964184 or rs139961185, respectively, before or after the 168 MB bp position, indicated by the vertical line. Full size image To investigate whether admixed ancestry confounds selection signal on chr11, we also performed the iHS analysis in all subjects homozygous for the Amerindian ancestry in the chr11 region ( n =1,217), as estimated by LAMP-LD. We observed iHS scores of 3.3 (rs609177) and 2.8 (rs111809212) in SIK3 . Interestingly, these variants are in LD with the Mexican-specific TG risk haplotype SNP rs139961185 in SIK3 , both resulting in R2>0.54 and D′>0.99 with rs139961185. Accordingly, they were also associated with high TGs when analysed in the entire Mexican TG case/control sample ( P =9.51 × 10 −7 and P =1.46 × 10 −10 ). These data show that the iHS scores remain large when the analysis is performed only on the Amerindian background, further supporting natural selection of SIK3 in Mexicans. Response to oral fat tolerance test in Mexicans To examine if the Mexican-specific SIK3 risk variant, rs139961185 affects postprandial TG metabolism, we carried out an oral fat tolerance test in a Mexican cohort. Briefly, the Mexican participants ate a fatty meal at the baseline and their TG levels were measured over a period of 8 h postprandially to calculate the postprandial TG response as an area under the curve (AUC) (see Methods for details of the diet study). 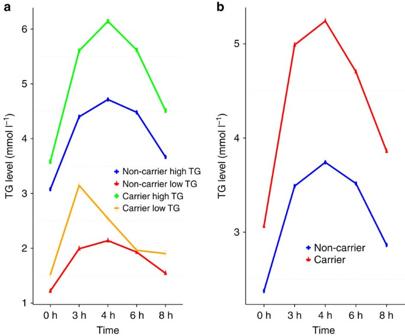Figure 5: Difference in postprandial TG clearance rate between rs139961185 risk allele carriers and non-carriers. The individuals carrying the rs139961185 risk allele inSIK3demonstrated a slower TG clearance rate (P=0.03 for AUC TG from linear regression) when compared with the non-carriers consistently (a) in Mexicans with low and high fasting TG levels at baseline and (b) in the combined study sample, suggesting thatSIK3is implicated for delayed postprandial TG clearance in Mexicans. There were 57 participants of which 3 and 9 were risk allele carriers (A/A and A/G) in the low and high TG group; and 17 and 28 were non-risk allele carriers (G/G) in the low and high TG group, respectively. Figure 5 demonstrates that both in the low TG (fasting baseline TG<1.69 mmol l −1 ) and high TG (fasting baseline TG>1.69 mmol l −1 ) groups ( Fig. 5a ) and in the combined Mexican study sample ( Fig. 5b ), the Mexican rs139961185 risk allele carriers consistently retained a significantly higher TG levels throughout the time course in contrast to non-carriers ( P =0.03 for TG AUC), suggesting that this TG-associated SIK3 risk variant may delay TG clearance after a fatty meal in Mexicans. Figure 5: Difference in postprandial TG clearance rate between rs139961185 risk allele carriers and non-carriers. The individuals carrying the rs139961185 risk allele in SIK3 demonstrated a slower TG clearance rate ( P =0.03 for AUC TG from linear regression) when compared with the non-carriers consistently ( a ) in Mexicans with low and high fasting TG levels at baseline and ( b ) in the combined study sample, suggesting that SIK3 is implicated for delayed postprandial TG clearance in Mexicans. There were 57 participants of which 3 and 9 were risk allele carriers (A/A and A/G) in the low and high TG group; and 17 and 28 were non-risk allele carriers (G/G) in the low and high TG group, respectively. Full size image Admixed populations provide unprecedented opportunities to understand human demographic history and genetic diversity, and moreover, to uncover variants of different ancestral origin and frequency that may contribute to variations in disease prevalence between populations [26] , [27] . However, genetic studies in recently admixed populations have proven difficult due to the confounding effects of population substructure and the reliance on an ancestral population reference panel that might not be readily available [15] , [16] . To this end, we designed a CPAS-GWAS approach that restricts GWAS to include only those variants that differ in frequency between the two ancestral populations. We performed the first CPAS-GWAS to discover Amerindian variants associated with dyslipidemia and obesity in Mexicans. Hypoalphaproteinemia, hypertriglyceridemia and hypercholesterolaemia are more prevalent in Amerindian-origin populations than in Europeans, with 60.5% Mexicans suffering from hypoalphaproteinemia (HDLC<1.03 mmol l −1 ); 43.6% from hypercholesterolaemia (TC>5.17 mmol l −1 ); and 31.5% from hypertriglyceridemia (TG>1.69 mmol l −1 ), respectively [1] , [2] , [5] , [28] , [29] . Clinical significance of dyslipidemia derives from the fact that patients with these lipid disorders are predisposed to CHD and often exhibit type 2 diabetes (T2D). CHD and T2D emerged as the two leading causes of death in Mexico in a recent national survey [30] , and more than 65% of the Mexican diabetics have hypertriglyceridemia [31] . Furthermore, recent evidence demonstrate a causal role of TGs in CHD [3] , [32] , [33] , [34] . Thus, it is critical to focus efforts and resources on the identification of the population-specific genetic components that make hypertriglyceridemia so prevalent in Mexicans. In contrast to other methods used to analyse admixed populations, CPAS-GWAS is able to achieve single-variant resolution uncovering susceptibility variants or their proxies instead of wider ancestry-enriched chromosomal regions identified using other approaches [15] , [16] . For example, our TG CPAS-GWAS identified eight Amerindian hypertriglyceridemia variants and one Amerindian-specific risk haplotype, of which all but one reside in genomic regions enriched for Amerindian ancestry in Mexican high TG cases as shown by local ancestry analysis. A two-step tree-based approach evaluating selection on a set of SNPs from several populations has previously been proposed that examines frequency difference among populations [35] . First, Bhatia et al . [35] built an unrooted tree utilizing Fst to identify divergence between populations followed by selection estimation at each marker common to all populations. To identify the potential traits under selection, they cross-referenced selected variants with GWAS catalogues. While CPAS and the tree-based method share similarity, they do not follow the same assumption and principle. CPAS does not assume variants to be under selection, rather we first screen for population-specific variants by comparing phenotypically matched distinct populations and then test their association with a trait directly. As a result, we can also identify population-enriched risk variants that correlate with a phenotype but are not necessarily under selection pressure, as is the case for instance with the LPL locus. Overall, our data demonstrate that CPAS-GWAS can effectively screen for ancestry-specific susceptibility variants in admixed populations. CPAS-GWAS is not restricted to a single admixed population or trait, and in fact, it can easily be tailored for other populations or diseases as shown by our qualitative TG and quantitative HDLC, TC and BMI CPAS-GWAS analyses. Moreover, CPAS-GWAS is not vulnerable to estimation of local ancestry that can be nontrivial if the appropriate parental populations are unknown or unavailable, as is often the case for admixed Latino populations [16] . Accordingly, false positives due to incorrect ancestry calculations are major concerns of local ancestry inference [15] , [16] . However, CPAS-GWAS does not face the same challenge as this step is eliminated. One limitation of the CPAS-GWAS approach is that its resolution and accuracy rely on the density of the genotyping arrays and the quality of imputation, but both will likely be circumvented in the near future as whole genome or exome sequencing become common practice as the price of sequencing continues to drop. We utilized Finns as surrogates of Europeans in CPAS, because Finns are the single largest population group investigated in extensive European lipid GWAS studies [11] , [13] , suggesting that Latino comparisons against Finns should sufficiently screen against the European lipid signals. Chromosome 11q23 harbours a well-known TG-associated APOA1C3A4A5 gene cluster, and the variant rs964184 has been implicated for TGs in multiple populations [8] , [9] , [10] , [11] , [12] , [13] , [14] . In this key TG region, CPAS-GWAS identified Amerindian TG risk variants and haplotype signatures, of which the most striking example is HT1 with zero frequency in Europeans and 20% frequency in Mexican TG cases. Of variants tagged by the haplotypes, rs11820589 and rs662799 explain ~6% of variability of TGs in Mexicans. Rs11820589 is in strong LD with a non-synonymous SNP (S19W), rs3135506, a known TG-increasing variant that resulted in a three-fold lower plasma Apo A-V levels when introduced in the mouse genome [24] . Rs662799, previously associated with both TGs and CHD [23] , resides in the promoter or enhancer region of APOA5 . It is worth noting that these TG risk variants rs3135506 and rs662799 are >2 and ~4 times more prevalent in the Mexican TG controls and Mexican TG cases than in the Finnish TG controls, respectively. APOA5 is a potent regulator of serum TG levels, as knockout mice lacking apoa5 have four times higher TG levels; mice expressing a human APOA5 transgene have one-third lower plasma TG levels; and overexpression of APOA5 reduces TG levels in mice [36] , [37] , [38] . In addition, APOA5 stimulates the LPL -mediated VLDL-TG hydrolysis via interaction with proteoglycan-bound LPL [38] , [39] . The variants rs662799 and rs3135506 likely affect the function of APOA5 , which in turn regulates LPL that is reflected as elevated TG levels in Mexicans. Targeted sequencing of the chr11q23 haplotype region that has substantial Amerindian ancestry in Mexican TG cases is bound to identify additional functional variants that influence TG levels in Amerindian-origin populations. We also identified two TG loci on chr8p21 and chr8p23 with a significant Amerindian ancestry in the Mexican TG cases. Rs79632214 is located downstream of the key TG gene, LPL , previously associated with TGs and CHD [11] , [40] , [41] . In Mexicans rs79632214 is in tight LD with rs328 (S474X), resulting in an early stop in LPL . Interestingly, our SKAT-C data implicated the presence of multiple Amerindian rare risk variants in the LPL region contributing significantly to TGs in Mexicans. Variant rs28680850 on chr8p21 is intergenic and the region has not previously been implicated for lipids in other populations. Our initial data show that this novel TG variant influences differential methylation of a CpG site, suggesting that allele-specific methylation contributes to the underlying biological mechanism. CPAS-GWAS also identified two novel replicated HDLC loci and one BMI locus that reside near or within genes that have never been associated with either trait in human. Interestingly, the new HDLC variant rs148533712 on chr15 is located in an intron of the retinoic acid RORA gene, and it is an independent signal of LIPC. RORA is a known transcriptional activator of APOA5 , APOA1 and APOC3 [42] , [43] , [44] , all residing in the Mexican risk haplotype region on chr11, suggesting distinct converging lipid pathways underlying dyslipidemia in Mexicans. At the chr20 BMI locus, protein phosphatase 1, regulatory subunit 3D ( PPP1R3D ) was recently identified for obesity in mice [45] . Thus, additional genes affecting BMI likely exist at this locus. To the best of our knowledge, we carried out the first study examining positive selection of GWAS loci for metabolic traits in an admixed population. TG is the most plausible trait under selection at these loci since our diet study implicates SIK3 in delayed TG clearance after a fatty meal; the chr11 locus displays the strongest association signal with TGs both in Mexicans and Europeans; and the novel chr8p23.3 region does not have significant associations with any other traits we tested ( P >0.0003). Furthermore, converging evidence from our selection analysis and diet study; TG and HDLC CPAS-GWAS; as well as a previous mouse model all support the role of SIK3 in metabolic functions. Interestingly, these Mexican-specific TG and HDLC CPAS variants in SIK3 are not present, and thus have not previously been identified in extensive European lipid GWAS studies [11] , [13] , suggesting that there are Amerindian-specific genetic lipid pathways involving SIK3 . Notably, recent data on a Sik3 knockout mouse identified SIK3 as a novel energy regulator, altering cholesterol and bile acid metabolism by coupling with retinoid metabolism [46] . We also searched the Gene Expression Omnibus [47] database at the NCBI and ArrayExpress [48] database at the European Bioinformatics Institute to verify that SIK3 is expressed in human liver and adipose tissues, the most relevant tissues in lipid metabolism. Furthermore, the iHS analysis suggests that SIK3 has been under positive selection pressure, pointing to an advantageous role for SIK3 in reproductive survival. However, whether selection pressure was acting on Amerindians prior to or after admixture requires further investigation. One possible explanation is that the ability to retain sufficiently high serum lipid levels could have contributed to the survival when resources were scarce during the early period of human habitation in the America continent. As a result, this genetic background was preferentially retained in the population. Additionally, in line with the selection results, our fatty diet study demonstrated that the Mexican-specific rs139961185 TG risk allele is significantly associated with delayed postprandial TG clearance in Mexicans, further supporting the role of SIK3 in TG metabolism and its candidacy for future functional studies. Individually, these findings do not stand alone as evidence of selection on TGs. However, taken together, they suggest that the SIK3 gene, associated with TGs in modern Mexicans, has undergone selection at some point during the Amerindian lineage. SIK3 may thus be a genetic responder to the Western diet that was recently introduced to Latinos, contributing to increased susceptibility to metabolic diseases in modern Mexicans. Additional future studies with whole-genome sequence data will help more comprehensively evaluate selection of lipid traits across the genome in Mexicans. In summary, we developed the CPAS-GWAS approach to uncover Amerindian variants in Mexicans that contribute to their greater susceptibility to dyslipidemia and obesity when compared with Europeans. Of the novel lipid genes we identified, RORA and SIK3 are of major interest. RORA is a transcriptional ligand-regulated mediator of multiple key lipid genes [42] , [43] , [44] , [45] . Furthermore, selective inhibition of the retinoic-acid-receptor-related orphan receptors via synthetic ligands has been suggested as a viable therapeutic approach for metabolic disorders [49] . Based on our findings from CPAS-GWAS, local ancestry, selection analysis, and oral fat tolerance test, we hypothesize that SIK3 may have played an important role in maintaining high plasma TG level that was historically critical for Amerindian survival but led to a higher rate of dyslipidemia and obesity in modern Hispanics after the adaption of Western diet. Our results suggest SIK3 as a strong candidate for future functional investigation to elucidate the molecular basis of the high prevalence of dyslipidemia in Mexicans. Human subjects A total of 19,273 participants from Finnish ( n =9,791) and Mexican ( n =9,482) cohorts were included in the study (see Supplementary Table 2 for clinical characteristics). All studies were approved by local research ethic committees: the Institutional Review Boards (IRB) of the Helsinki, Turku and Tampere University Hospitals; IRB of the National Institute for Health and Welfare; IRB of the Instituto Nacional de Ciencias Médicas y Nutrición, Salvador Zubiran; and IRB of UCLA), and all participants gave informed consent. We screened six Finnish population-based cohorts with GWAS data available [50] , [51] , [52] (total n =14,217) for individuals with low serum TG levels (TGs<1.69 mmol l −1 ) and not taking lipid-lowering medication. Fasting TG values were used to determine the low TG status, except for the FINRISK cohort. However, since non-fasting does increase and does not decrease serum TG levels, the use of non-fasting TGs in that cohort should not influence the results. A subset of 9,791 Finnish individuals with low TGs were included in the cross-population screening step from the Northern Finland Birth Cohort 1966 (NFBC66) ( n =4,427), the Cardiovascular Risk in Young Finns Study ( n =1,428), Helsinki Birth Cohort Study ( n =991), Health2000 GenMets Study ( n =1,301), FinnTwin12 and FinnTwin16 cohort studies (Twins) ( n =421; one randomly selected twin in each twin pair was selected to investigate only unrelated subjects), and FINRISK ( n =1,223). The Finnish GWAS data on the NFBC1966 Study has been previously deposited in the NIH dbGAP data repository under the accession code phs000276.v1.p1. Two Mexican cohorts ascertained for hypertriglyceridemia [14] or T2D [53] were combined and screened for low TG controls (fasting TGs<1.69 mmol l −1 ) ( n =1,645) and high TG cases (fasting TGs>2.26 mmol l −1 ) ( n =1,678), excluding individuals on lipid-lowering medication. The Mexican participants were recruited at the Instituto Nacional de Ciencias Médicas y Nutrición Salvador Zubirán, Mexico City. In the replication stage, we investigated 6,159 additional Mexican individuals for replication of 15 SNPs using the same criteria for the hypertriglyceridemia status as in the cross-population allele screen, which resulted in 2,129 high TG cases, 2,985 low TG controls and 903 family members from 73 Mexican dyslipidemic families [14] , [54] , [55] . To utilize all individuals with lipid phenotypes available in these cohorts ( n =6,159), we also analysed log-transformed serum TGs as a quantitative trait. Serum TGs, HDLC and TC were measured using enzymatic and enzymatic colorimetric methods with commercial reagents in the Finnish and Mexican cohorts [50] , [51] , [52] , [53] , [54] . The cut-points for TG cases (TGs>2.26 mmol l −1 ) and TG controls (TGs<1.69 mmol l −1 ) are based on the American Heart Association TG guidelines. The general population means of HDLC, TC and BMI in Finns and Mexicans were used as cut-points in the two populations for the CPAS stage to screen for controls. The thresholds of the three traits for controls in Finns and Mexicans were as follows: HDLC>1.15 mmol l −1 and HDLC>1.54 mmol l −1 ; TC<5.17 mmol l −1 for both populations; and BMI <25 kg m −2 and BMI<27 kg m −2 , respectively. The Mexican participants ( n =57) included in the fatty meal diet study were recruited at the Instituto Nacional de Ciencias Médicas y Nutrición Salvador Zubirán, Mexico City. Genotyping and imputation In the CPAS, Illumina genotyping platforms were used for all cohorts, as described in detail previously [14] , [50] , [51] , [52] . The NFBC cohorts were genotyped with the HumanHap CNV 370k array: GenMets and FINRISK with the HumanHap 610 k array: and Young Finns Study, Helsinki Birth Cohort Study and Twins with the HumanHap 670 k array, respectively. The Mexican cohorts were genotyped using Human 610 BeadChip and Human Omni 2.5 BeadChip array, respectively. Genotype quality control was performed on each cohort separately using the following inclusion criteria: SNP and sample genotyping success rate ⩾ 95%, MAF ⩾ 1%, Hardy–Weinberg equilibrium (HWE) P ⩾ 1 × 10 −6 , and individual heterozygosity rate <4s.d. Samples with gender discrepancies or closely related individuals were removed. In the replication stage, SNPs were genotyped using Sequenom and TaqMan platform. These SNPs had a genotype call rate ⩾ 90%, and they passed a Bonferroni corrected HWE P -value>0.05 for the number of tested SNPs. In addition, the family data were checked for Mendelian errors using the Mendel [56] mistyping option. Imputation was carried out separately in Mexicans and Finns. To reduce imputation runtime, we first pre-phased the Mexican and Finnish cohorts separately using SHAPEIT with the 1000 Genomes Project reference panel [57] , [58] . Subsequently, imputation was carried out using IMPUTE2 utilizing the 1000 Genomes Project reference panel as well [59] , [60] . Following the IMPUTE2 guideline and results from a previous study, we employed a cosmopolitan imputation strategy that included all populations from the 1000 Genomes Project to maximize accuracy and the number of imputed SNPs [16] , [61] . Imputed data were filtered using the following quality control criteria: info ⩾ 0.8, probability ⩾ 0.9, MAF ⩾ 1% and HWE ( P >0.0001). Bisulphite pyrosequencing The methylation status of the CpG site containing the SNP, rs28680850, was measured using bisulphite pyrosequencing with custom-designed kit from EpigenDx according to the standard protocol for bisulphite treatment and pyrosequencing by the manufacturer. Association analyses Association testing at the CPAS step and the subsequent GWAS was carried out for the binary TGs status with logistic regression using an additive genetic model, including age, sex and BMI as covariates to control for their potential confounding effects on serum TGs at the allele screen step. For the quantitative CPAS-GWAS analysis of HDLC and TC levels, HDLC and TC levels were first log-transformed to approximate normal distribution, and multiple linear regression was used with age, sex, BMI, global ancestry estimates and the high TG status as covariates. For the quantitative CPAS-GWAS analysis of BMI, age and sex were used as covariates in linear regression, as no inflation was observed ( Supplementary Figs 11–14 ). Imputed SNPs were analysed using SNPTEST v2.4 (ref. 62 ) and the score method was used to incorporate the imputation uncertainties into the regression model. Redundant SNPs with a MAF>5% were pruned based on LD with R 2 ⩾ 0.5 in Mexican controls. In the CPAS step for qualitative TGs, a Bonferroni correction for 1,584,455 tested SNPs ( P <3.16 × 10 −8 ) was used to identify variants that have different allele frequencies in Mexicans and Finns, resulting in 967,056 SNPs that were significantly different and carried forward to the TG GWAS ( Supplementary Fig. 1 ). The set of SNPs ( n =694,185) that were variable in Mexicans but were monomorphic in the Finnish cohorts were also included in the GWAS to capture additional Amerindian-specific TG-associated variants. A total of 1,661,241 SNPs were analysed in the TG GWAS ( Supplementary Fig. 1 ). We also performed CPAS for the three additional traits, HDLC, TC and BMI in a similar way ( Table 2 ). The quantile–quantile plots ( Supplementary Figs. 11–14 ) of the all GWAS results with the CPAS SNPs demonstrate that most of the distribution behaves as the expected null, ruling out major confounders. Haplotype logistic regression, step-wise logistic regression and McKelvey and Zavoina pseudo-R 2 analysis, and Mantel–Haenszel test were all performed in R statistical package ( http://www.r-project.org/ ). Conditional association analysis on rs964184 was carried out using SNPTEST2.4 with the SNP genotype as a covariate. Association analyses of the 15 TG SNPs genotyped in the replication stage were performed employing the same logistic regression model as in the GWAS using PLINKv1.08 package [63] . In the replication stage, we also performed a quantitative trait analysis on log-transformed TG levels including sex and age as covariates using PLINK. For the two HDLC SNPs, linear regression was carried out using PLINK as well, including sex, age, BMI, high TG status and global ancestry as covariates. Part of the independent cohort ( n =2,121) was used for HDLC replication as these samples have global ancestry estimates available. The family cohort was analysed using the quantitative trait locus association option of Mendel [64] . After taking into account multiple testing using Bonferroni correction, P -values of 0.0033 (15 tested SNPs), 0.025 (two tested SNPs) and 0.05 (one tested SNP) were considered as statistically significant in the replication stage for TG, HDLC and BMI SNPs, respectively, when combining the P -values of the two replication cohorts by weighting by sample size using METAL [20] or the subset of independent cohort for HDLC. Analysis of combined rare and common variant effects was carried out using SKAT-C implemented in R with a window size of 50 kb and a sliding window of 40 kb. To increase the number of rare variants in SKAT, we used a 5% frequency cutoff. Alternatively, we also calculated the rare variant frequency as where N is the sample size ( N =3,701). Local ancestry inference To investigate whether variants identified utilizing the cross-population allele screen approach reside in chromosomal genomic regions enriched for Amerindian ancestry in the Mexican high TG cases, we carried out local ancestry estimation utilizing Local Ancestry in adMixed Populations using LD (LAMP-LD) [17] . A three-population mixed model was assumed to estimate proportions of the three ancestral populations (European, Amerindian and African) in the modern Mexicans [65] . The parental population reference panels were constructed from individuals in the Genetics of Asthma in Latino Americans [66] study as described in detail previously [18] and LAMP-LD was run with default parameters, window size 300 and 15 hidden Markov models states, on each chromosome separately. To identify Amerindian enriched regions associating with TG, the standard scores of the difference in local Amerindian ancestry between the Mexican TG cases and controls were calculated for each region. A significance threshold of z -score>2 was used to call ancestral enrichment. To calculate the percent difference between cases and controls for each ancestral population, the proportion of all parental populations was estimated for every window in cases and controls separately, and the difference was calculated between the cases and controls for individual ancestry. Analysis of positive natural selection To examine if the 8p21, 8p23.3 and chr11q23 TG risk regions have undergone partial selective sweeps, we searched for haplotypes that were unusually long, given the frequency of the focal variant [67] . Specifically, we first estimated extended haplotype homozygosity using the ‘rehh’ R package [68] . Next, we calculated the integrated extended haplotype homozygosity for both ancestral and derived alleles for each genotyped SNP with MAF>5% and then calculated the standardized natural log ratio of integrated extended haplotype homozygosity between ancestral and derived alleles (iHS) [25] . Similarly, we also calculated the iHS scores for imputed variants only in the two chr8 TG risk regions and chr11 risk haplotype region due to computing time. All calculations were performed in the entire Mexican GWAS study sample and including all variants (MAF>5%) without any ascertainment or CPAS screening to avoid a potential bias. We used the top 1% chromosome-wide absolute iHS (|iHS|) score (>2.56) as a cutoff to identify SNPs showing extremely large values of iHS. Fatty meal study in Mexican cohort The 57 Mexican participants underwent an oral fat tolerance test after a 12-hour overnight fast. The fatty meal contained 1,000 kcal; 72 g fat (saturated fat 65%, monounsaturated fat 30%, polyunsaturated fat 5%) with polyunsaturated:saturated fat ratio of 0.08, 490 mg cholesterol, 50 g carbohydrate and 38 g protein, as described in detail earlier [69] . In this diet study, blood samples were drawn at the baseline and at 3, 4, 6 and 8 h postprandially. Postprandial TG response was calculated as an AUC, as described in detail earlier [70] . The intronic SIK3 variant rs139961185 was genotyped in the 57 participants of which 20 had fasting TG levels <1.7 mmol l −1 at the baseline (the low TG group) and 37 had fasting TG levels >1.7 mmol l −1 at the baseline (the high TG group). To test for association between rs139961185 and postprandial TG clearance rate, a linear regression for TG AUC was performed using an additive genetic model and adjusting for the baseline TG status. How to cite this article: Ko, A. et al . Amerindian-specific regions under positive selection harbour new lipid variants in Latinos. Nat. Commun. 5:3983 doi: 10.1038/ncomms4983 (2014).